Plasmofluidic single-molecule surface-enhanced Raman scattering from dynamic assembly of plasmonic nanoparticles Single-molecule surface-enhanced Raman scattering (SM-SERS) is one of the vital applications of plasmonic nanoparticles. The SM-SERS sensitivity critically depends on plasmonic hot-spots created at the vicinity of such nanoparticles. In conventional fluid-phase SM-SERS experiments, plasmonic hot-spots are facilitated by chemical aggregation of nanoparticles. Such aggregation is usually irreversible, and hence, nanoparticles cannot be re-dispersed in the fluid for further use. Here, we show how to combine SM-SERS with plasmon polariton-assisted, reversible assembly of plasmonic nanoparticles at an unstructured metal–fluid interface. One of the unique features of our method is that we use a single evanescent-wave optical excitation for nanoparticle assembly, manipulation and SM-SERS measurements. Furthermore, by utilizing dual excitation of plasmons at metal–fluid interface, we create interacting assemblies of metal nanoparticles, which may be further harnessed in dynamic lithography of dispersed nanostructures. Our work will have implications in realizing optically addressable, plasmofluidic, single-molecule detection platforms. Interaction of light with nanoscale matter at sub-wavelength regimes has gained attention in various branches of science and technology. The significance of this interaction is driven by the fact that quantum systems, such as atoms, molecules, quantum dots and their varieties, can be individually coupled to electromagnetic fields at the nanoscale [1] , [2] , [3] , [4] , [5] . Studying molecules at single copy-limit not only has tremendous implications in chemical and biological sensing [2] , [6] , [7] , but also can lead to new physical insights about molecules that are not evident when their respective ensembles are interrogated [8] , [9] , [10] . Controlling electromagnetic fields at nanoscale is one of the important tasks of nanophotonics, and to serve this purpose plasmons, which are charge density oscillations at metal dielectric interface, have been utilized extensively [11] , [12] , [13] . Plasmons are usually produced in two major varieties: one is the localized surface plasmons (LSPs) facilitated by metal nanoparticles and junctions between nanostructures [14] , and the other is the surface plasmon polaritons (SPPs) that are usually propagating in nature, and can be produced on a variety of platforms such as films, nanowires etc [15] . There are various applications of plasmons [16] , [17] , [18] , [19] , [20] of which two are directly relevant to this study: solution-phase single-molecule surface-enhanced Raman scattering (SM-SERS) and trapping of nano-scale objects in plasmofluidic field (that is, plasmonic field in fluidic environment). The SM-SERS was first achieved in 1997 (refs 21 , 22 ), and ever since it has emerged as one of the important nanoscale spectroscopy techniques to interrogate both molecules and localized optical fields [23] , [24] , [25] , [26] , [27] , [28] , [29] . Plasmon-assisted optical trapping [30] , [31] , [32] , [33] , [34] can be utilized to trap and manipulate micro- and nano-scale objects at metal–fluid interface [35] , [36] , [37] , [38] , [39] , [40] , [41] with laser powers significantly lower than the conventional optical trapping. One of the objectives of this work was to integrate SM-SERS with plasmon-assisted assembly of nanoparticles in solution. This integration is advantageous, especially in the context of optofluidics, for the following reason. In most of the solution-phase SM-SERS experiments [23] , [42] , [43] , [44] , the plasmonic hot spots are facilitated by adding chemical aggregating agents such as NaCl or KCl. These chemicals agglomerate the nanoparticles irreversibly, and hence the aggregates cannot be further used as uniformly dispersed, plasmonic nanoscale entities. Also, such procedure of aggregation is not conducive for micro/nano-fluidic environments, where a relatively small aggregate can block the flow of the liquid. Therefore, there is an imperative need to temporarily assemble nanoparticles in a controlled way, and re-disperse them back in the fluid after SM-SERS interrogation. In this paper, we show how to combine SM-SERS with plasmon-assisted assembly and manipulation of metal nanoparticles without the use of aggregating agents. Importantly, a single evanescent-wave optical excitation was used to achieve both plasmonic assembly and SM-SERS, simultaneously. To best of our knowledge, this is the first report on solution-phase SM-SERS experiments on dynamic assembly of metal nanoparticles by evanescent-wave excitation of plasmons. By harnessing the optical fields created by SPPs in a metal film, we create large-area assembly of metal nanoparticles, and further use the combination of SPP and LSP fields to capture SM-SERS signatures at metal–fluid interface. In addition to this, we show the potential of our method to achieve dynamic, large-area lithography of nanoparticles at metal–fluid interface by using dual-optical excitation in total-internal reflection (TIR) geometry. Combining plasmonic assembly with SERS microscopy We first addressed the issue of how to effectively use a single evanescent-wave optical excitation at metal–fluid interface to simultaneously assemble plasmonic nanoparticles and perform Raman scattering. For this, we utilized TIR-based plasmonic excitation of an unstructured metal film in Kretschmann geometry. This plasmon-polariton excitation created an optical potential, which was further utilized to assemble and manipulate nanoparticles. Importantly, the same TIR illumination was also utilized for exciting the Raman scattering from the assembled nanoparticles. 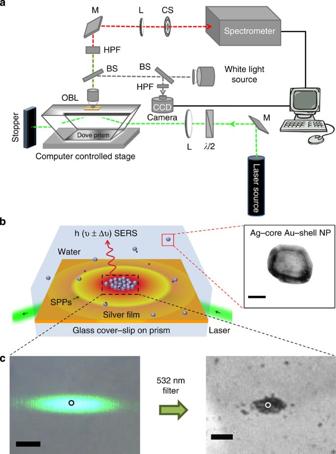Figure 1: SERS microscopy combined with plasmon-assisted assembly of nanoparticles. (a) Optical set-up of confocal Raman detection microscope coupled with Dove-prism-based plasmon excitation. (b) Schematic illustration of the simultaneous plasmonic assembly of nanoparticles and SERS. Black arrows indicate the direction of 532 nm laser (green beam) used for SPP excitation of the metal film deposited over glass coverslip. Grey spheres are the metal nanoparticles dispersed in the water medium and red dots indicate the SERS-active molecules. Inset on the right shows the TEM image of Ag core-Au shell nanoparticle used in this experiement. Scale bar is 20 nm. (c) On the left is an unfiltered optical bright-field image of 532 nm elliptical excitation on the metal film; the right side image shows the plasmon-assisted assembly of nanoparticles in the excitation region (532 nm rejected using filter). The open circles incindicates the area from which SERS signals were collected. Scale bar is 80 μm. BS, beam splitter; CCD, charged-coupled device; CS, confocal slit; HPF, high pass filter; L, lens; M, mirror; OBL, objective lens; λ/2, half wave plate. Figure 1a shows the optical schematic of the set-up used for plasmon-assisted assembly of metal nanoparticles and SM-SERS measurements. We used a Dove prism (N-BK7, refractive index=1.519), on to which a silver-coated glass coverslip was adhered through an optically matched oil. The thickness of the metal film was 40±5 nm. The excitation source was a 532-nm continuous-wave frequency-doubled Nd:YAG laser (power up to 200 mW), which was p-polarized by a λ /2 plate and routed into the prism for TIR by weakly focusing lens L (focal length=150 mm). The angle of incidence at the interface was 76.7° from the normal to the surface, which was close to the TIR angle of Ag–water interface (see Supplementary Fig. 1 ). The optical image and the Raman scattered signal from the metal–water interface was collected via an objective lens (OBL). For conventional optical imaging, a × 4, 0.13 numerical aperture (NA) lens was used, whereas for the SM-SERS measurements, a water immersion OBL ( × 60, 1.0 NA) was used. The captured light was routed towards the camera or into a high resolution, confocal Raman spectrometer (LabRam HR, 789 mm focal length, pinhole size=400 μm). The p-polarized Gaussian excitation beam creates an elliptical projection upon TIR at the metallic surface, which was imaged in Fig. 1c . This particular excitation profile acts as an optical potential, which was harnessed for plasmofluidic trapping and SM-SERS measurements. Upon introducing bimetallic core-shell nanoparticle solution (80 μl) on to the Ag surface, the nanoparticles slowly (within 15 min) assembled at the location of the elliptical spot. One such assembly of nanoparticles is shown in Fig. 1c by filtering the incident laser beam. The open circle shown in Fig. 1c is the location from where the confocal Raman signals were captured. Figure 1: SERS microscopy combined with plasmon-assisted assembly of nanoparticles. ( a ) Optical set-up of confocal Raman detection microscope coupled with Dove-prism-based plasmon excitation. ( b ) Schematic illustration of the simultaneous plasmonic assembly of nanoparticles and SERS. Black arrows indicate the direction of 532 nm laser (green beam) used for SPP excitation of the metal film deposited over glass coverslip. Grey spheres are the metal nanoparticles dispersed in the water medium and red dots indicate the SERS-active molecules. Inset on the right shows the TEM image of Ag core-Au shell nanoparticle used in this experiement. Scale bar is 20 nm. ( c ) On the left is an unfiltered optical bright-field image of 532 nm elliptical excitation on the metal film; the right side image shows the plasmon-assisted assembly of nanoparticles in the excitation region (532 nm rejected using filter). The open circles in c indicates the area from which SERS signals were collected. Scale bar is 80 μm. BS, beam splitter; CCD, charged-coupled device; CS, confocal slit; HPF, high pass filter; L, lens; M, mirror; OBL, objective lens; λ/2, half wave plate. Full size image Choice of the metal films and nanoparticles Trapping of plasmonic nanoparticles on metal film is extremely sensitive to three parameters: plasmon resonance of the nanoparticles, SPP resonance of the film and excitation wavelength (see Supplementary Figs 2 and 3 for the data on resonances of various metal films and nanoparticles). We found that if the resonance of nanoparticles has a large overlap with the excitation wavelength, as in case of Au nanoparticles at 532 nm, then nanoparticles usually escaped from the trap, and were not suitable for our experiments. Such propulsion of Au nanoparticles in SPP field has also been reported by various researchers [45] , [46] , [47] , [48] . As an alternate to Au nanoparticles, we used Ag-core Au-shell (Ag@Au) nanoparticles. Recently, we have shown [44] that Ag@Au nanoparticle architectures are excellent substrates for SM-SERS experiments at visible frequencies. There are at least three advantages [49] of using such nanoparticles: (1) they facilitate optical near-fields comparable to Ag nanoparticle and better than Au nanoparticle; (2) by varying the thickness of the gold shell, one can systematically tune the plasmon resonance from visible to infra-red wavelength; (3) as these particles have gold shell, they provide biocompatibility [49] and stability compared with Ag nanoparticles. With this hindsight, we tuned the Au shell-thickness of Ag@Au nanoparticle such that we obtained a plasmon resonance at 490 nm. This value was slightly off-resonance from the 532 nm excitation and hence suitable for both plasmonic assembly and SM-SERS experiments. Also, for the Ag film–water interface, the SPR resonance wavelength was found to be 500 nm, which was again off-resonance from our 532 excitation. Taking all the resonances and other advantages into consideration, we found Ag@Au nanoparticle suitable for both plasmonic assembly and SM-SERS experiments. 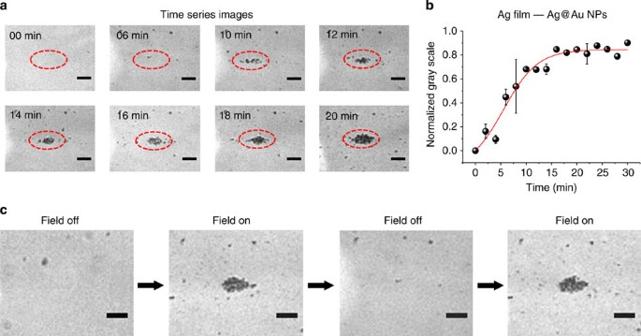Figure 2: Plasmon-assisted assembly of nanoparticles at metal–fluid interface. (a) Time series images of gradual-accumulation of Ag@Au nanoparticles on silver-film in evanescent optical field indicated by dotted-ellipse in red (seeSupplementary Movies 1 and 2). (b) Variation of particle density in the above-mentioned field as a function of time, extracted from the images. Solid red-line represents the least-square Boltzmann fit to the experimental data. Error bars on the experimental data points represent the variation (standard deviation) in determining the grey scale values across the optical images obtained throughout the experiment. (c) Optical bright-field images showing capability to repeat the assembly and release of nanoparticles in the presence and absence of plasmonic field at metal–fluid interface. Scale bar is 80 μm for all figures. Assembly of Ag@Au nanoparticle in plasmofluidic field Figure 2a shows the time series images of the assembled Ag@Au nanoparticles on a metal film in the presence of p-polarized evanescent-wave excitation (see Supplementary Movies 1 and 2 ). We observed a gradual aggregation of nanoparticle spanning over a time period of 30 min. Between 06 and 16 min, there was a steady increase in the number of nanoparticles assembled in the illuminated spot, but after 20 min, we found that the number of nanoparticles in the illuminated region reached a saturation point in time, and thereafter the aggregate reached a steady state. Figure 2: Plasmon-assisted assembly of nanoparticles at metal–fluid interface. ( a ) Time series images of gradual-accumulation of Ag@Au nanoparticles on silver-film in evanescent optical field indicated by dotted-ellipse in red (see Supplementary Movies 1 and 2 ). ( b ) Variation of particle density in the above-mentioned field as a function of time, extracted from the images. Solid red-line represents the least-square Boltzmann fit to the experimental data. Error bars on the experimental data points represent the variation (standard deviation) in determining the grey scale values across the optical images obtained throughout the experiment. ( c ) Optical bright-field images showing capability to repeat the assembly and release of nanoparticles in the presence and absence of plasmonic field at metal–fluid interface. Scale bar is 80 μm for all figures. Full size image Figure 2b shows the aggregate-growth kinetics of the nanoparticles in the dotted ellipse region. We captured the scattering intensity coming out of the elliptical region as a function of time, and the points in Fig. 2b shows the experimental data. The experimental growth kinetics data fitted well to a least-square Boltzmann equation (see Supplementary Note 1 for details). The accumulation of nanoparticles in the illuminated region was mainly due to the combination of fluid convection and SPP forces experienced by the nanoparticles. Similar kind of plasmofluidic assembly of dielectric microspheres on a gold nano-film has been reported by Garcés-Chávez et al. [35] The excitation of SPP on the film creates a gradient of temperature just above the illuminated region. The temperature distribution in the surrounding water medium is governed by the following equation [50] : where v(r,t) is the fluid velocity and ∇ . ( T v) is the nonlinear convective term. κ , ρ , c are the thermal conductivity, mass density and specific heat capacity of water at constant pressure, respectively. The temperature gradient creates convection in the fluid, and the nanoparticles move from the cooler region of the fluid into the hotter region, that is, towards the illuminated spot. Furthermore, the same convection current will try to drive the nanoparticles away from the hotter region, but the gradient force of SPP holds them back from escaping out, thereby trapping them at illuminated spot. It is to be noted that the LSP resonance of plasmonic nanoparticles also has an important role in this assembly. Trapping was feasible only when LSP resonance wavelength of nanoparticles was far from the excitation wavelength (532 nm). Apart from Ag@Au nanoparticles, we tested this hypothesis for Ag nanoparticles (420 nm resonance), and found excellent trapping capability. Interestingly, Ag nanoparticles assembled in the trap at a faster rate compared with Ag@Au nanoparticles (see Supplementary Fig. 4 ). Furthermore, we tested the reversibility of the nanoparticle assembly, by switching-off the evanescent-field excitation and later switched it back after a few minutes. Figure 2c shows the optical images of two such cycles of reversible assembly of Ag@Au nanoparticles, where the excitation fields were alternately switched on and off. We tested this process over multiple cycles (at least five times) and we found excellent consistency in terms of reversible assembly of nanoparticles at the illuminated location. SM-SERS from plasmon-assisted assembly of Ag@Au nanoparticles As many nanoparticles are packed into an assembly on the metal surface, one would expect multiple plasmonic hot spots in this confinement. Such hot spots are ideal for SERS experiments. [23] , [51] . Furthermore, the same optical excitation that is trapping these nanoparticles should also be able to excite SERS signatures of the molecules in the hot spot. Can these hot spots be sensitive enough to detect single-molecule Raman signatures? To answer this question, we employ bi-analyte SM-SERS method developed by Etchegoin and Ru [42] , [52] . This technique is based on spectroscopic contrast between two different kinds of SERS-active molecules, and importantly, does not rely on the ratio of number of molecules to the nanoparticles used in the experiments. From a large data set of SERS experiment, reliable single-molecule signatures can be extracted by rigorous statistical analysis based on modified principal component analysis (MPCA) [51] , [52] . The two molecules used for our experiments were nile blue (NB) and rhodamine 6G (R6G) at 5 nM concentration. For SM-SERS experiments, we choose 592 and 615 cm −1 Raman modes of NB and R6G, respectively. 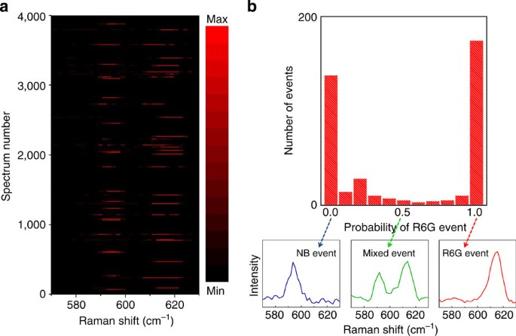Figure 3: Single-molecule SERS from the assembled Ag@Au nanoparticles. (a) Bi-analyte (nile blue (NB) and rhodamin6G (R6G)) SERS time-series spectra recorded from the open circle region shown inFig. 1c. The concentration of both the molecules was 5 nM. For modified principal component analysis (MPCA) analysis, 592 cm−1modes of NB and 615 cm−1mode of R6G were considered. 4,000 spectra (out of 7,000) have been displayed to show spectral fluctuation of single molecules in plasmonic field. Signal acquisition time was 0.1 s. All the data were collected using 532 nm evanescent excitation wavelength (20 mW power before entering the prism). (b) Single-molecule probability histogram derived from MPCA. Maximum event at 1 and 0 of abscissa confirms single-molecule SERS signal from R6G and NB, respectively. The inset shows spectral signatures for three different probabilities. Figure 3a shows time evolution of bi-analyte SM-SERS signal captured from the plasmofluidic trap of core-shell nanoparticles (see the open circle in Fig. 1c ). The total number of spectra collected was 7,000, the acquisition time for each spectrum was 0.1 s and the dwell time between consecutive accumulations was 1 s. We further processed this data using MPCA [52] to find the principal eigenvalues of the signals generated. All the details of the MPCA analysis can be found in the Supplementary Fig. 5 . The results of the MPCA analysis are shown in Fig. 3b , where the probability of single-molecule signature is plotted in the form of a histogram, and accompanying them are the relevant bi-analyte spectra for three different probabilities of single-molecule events (0 corresponds to single NB event, 0.5 for mixed event and 1 for single R6G event; the probability for detection of R6G single molecule is slightly greater than NB because electronic resonance of R6G is closer to 532 nm excitation).The histogram clearly indicates a large probability of single R6G and single NB molecules’ spectral signatures arising from the plasmofluidic trap of nanoparticles. These data are the central results of this paper. We emphasize that the SM-SERS excitation is arising from the same source, which is assisting us in trapping the nanoparticles. To best of our knowledge, this is the first report where both plasmofluidic assembly and SM-SERS have been concomitantly achieved using a single evanescent-wave excitation. Thus, our method not only creates multiple plasmonic hot spots in a nanoparticle assembly but also probes the single-molecule spectral signatures simultaneously. Figure 3: Single-molecule SERS from the assembled Ag@Au nanoparticles. ( a ) Bi-analyte (nile blue (NB) and rhodamin6G (R6G)) SERS time-series spectra recorded from the open circle region shown in Fig. 1c . The concentration of both the molecules was 5 nM. For modified principal component analysis (MPCA) analysis, 592 cm −1 modes of NB and 615 cm −1 mode of R6G were considered. 4,000 spectra (out of 7,000) have been displayed to show spectral fluctuation of single molecules in plasmonic field. Signal acquisition time was 0.1 s. All the data were collected using 532 nm evanescent excitation wavelength (20 mW power before entering the prism). ( b ) Single-molecule probability histogram derived from MPCA. Maximum event at 1 and 0 of abscissa confirms single-molecule SERS signal from R6G and NB, respectively. The inset shows spectral signatures for three different probabilities. Full size image Although we have shown the spectroscopic signature of SM-SERS in dynamic assembly of plasmonic nanoparticles, it is to be noted that we are still constrained by the far-field diffraction limit of our microscope. This means that we do not detect individual entities of single molecules in the plasmofluidic trap of nanoparticles, but we probe only the SM-SERS signatures of a few molecules in the plasmofluidic trap. In our experimental configuration, there are two kinds of plasmonic fields: one is the SPP field created by the metal film and the other is the LSPs of the nanoparticles. Importantly, the SPPs of the film can couple to the LSPs of the nanoparticles [53] , [54] , [55] , [56] , [57] , [58] , [59] , [60] . This combination of the SPP and LSP can facilitate large electric fields thereby creating plasmonic hot spots at two locations: junction between film and nanoparticles, and the junction between individual nanoparticles. Furthermore, nanoparticles assemble in both horizontal and vertical direction, leading to multiple hot spots in the illuminated region of metal–fluid interface. We further corroborated this hypothesis with 3D-finite difference time domain calculations (see Supplementary Fig. 6 and Supplementary note 2 ), which indicated near-field enhancement to arise due to film–particle coupling and particle–particle coupling. Such multiple hot spots at metal–fluid interface can facilitate large-scale enhancement, and our experimental result of single-molecule spectroscopic detection is one such important consequence due to the near-field coupling between the molecules and nanoparticles. Plasmon-assisted manipulation of Ag@Au nanoparticle assembly Having shown the capability to perform SM-SERS at metal–fluid interface, we asked whether we can systematically manipulate the trapped assembly of nanoparticles, such that they can be utilized as optically addressable, SM-SERS substrate in a fluid. To answer this, we probed the effect of moving the elliptical excitation beam on the plasmonic nanoparticle assembly. 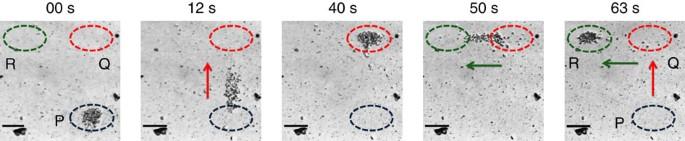Figure 4: Plasmon-assisted manipulation of Ag@Au nanoparticle assembly at metal–fluid interface. Time series images showing transportation of nanoparticle assembly from initially trapped area P to final area R via point Q (seeSupplementary Movie 3). The manipulation involves a right-angled turn, which was achieved by careful movement of evanescent excitation beam. The assembly of nanoparticles were accurately transported over a distance of 300 μm within few seconds. Note that the manipulation was achieved on an unstructured metal–fluid interface. Scale bar is 80 μm. Figure 4 shows the optical images (time series) of plasmonic nanoparticle transport at metal–fluid interface (see Supplementary Movie 3 ). The different locations—P, Q and R in Fig. 4 —indicate the three parking points of elliptical excitation beam. We first started with a plasmonic assembly at P. Next, we moved the excitation beam to the location Q, and after a few seconds we observed gradual migration of the plasmonic nanoparticles into new location, Q. About 40 s later, we changed the location of optical excitation from Q to R, and within a few seconds, the nanoparticle assembly followed the excitation beam. This experiment revealed two important aspects of the trap: (1) capability to accurately manipulate a large assembly of nanoparticles in fluid by plasmon-assisted excitation without structuring the metal surface , and (2) the robustness to overcome any Brownian drag forces during the movement of the assembly. These advantages can be further harnessed in plasmon-assisted micro- and nano-fluidics with an added capability of single-molecule detection sensitivity. Figure 4: Plasmon-assisted manipulation of Ag@Au nanoparticle assembly at metal–fluid interface. Time series images showing transportation of nanoparticle assembly from initially trapped area P to final area R via point Q (see Supplementary Movie 3 ). The manipulation involves a right-angled turn, which was achieved by careful movement of evanescent excitation beam. The assembly of nanoparticles were accurately transported over a distance of 300 μm within few seconds. Note that the manipulation was achieved on an unstructured metal–fluid interface. Scale bar is 80 μm. Full size image It is to be noted that our methodology is versatile and can be applied to different combinations of metal films and plasmonic nanoparticles. Table 1 compares a variety of such combinations for 532 nm excitation. Parameters such as nanoparticle assembly time, assembly size and the SERS signal retrieved from such assemblies are compared. Specifically for SM-SERS studies, we found Ag@Au nanoparticles and Ag nanoparticles on Ag film to be suitable. Also, other combinations of film and particles can be harnessed for conventional SERS studies. Table 1 Comparison between various combinations of metal films and nanoparticles. Full size table Towards dynamic lithography of nanoparticles Can we utilize our method in dynamic lithography of dispersed nanoparticles at metal–fluid interface, such that they can be temporarily assembled in a specific geometry and further re-dispersed in the fluid? To answer this question, we performed experiments with Ag nanoparticle on Au film (combination 4 in Table 1 ) with a dual 532-nm evanescent-wave excitation in counter-propagating geometry. 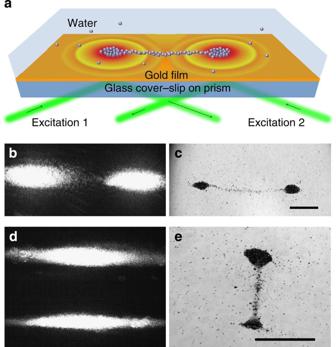Figure 5: Interaction between dynamic assemblies of plasmonic nanoparticles at metal–fluid interface. (a) Schematic representation of dual assembly of Ag nanoparticles on Au film coupled to a prism: green lines are the two laser beams of 532 nm introduced at two opposite ends of the prism. Black arrows indicate the direction of the laser beams (seeSupplementary Movie 4). Optical images of dual laser excitation inbcollinear geometry with opposite k-vectors and (d) anti-parallel geometries with opposite k-vectors. (c) and (e) are optical images (532 nm-rejected) of Ag nanoparticles assembly due to excitation in shown inbandd, respectively. A thin line of nanoparticles bridging the two assemblies is evident. Note that all these assemblies are at metal–fluid interface, and hence can be further manipulated to achieve dynamic lithography. Scale bar, 100 μm for both (c) and (e). Figure 5a shows the optical schematic of dual-excitation trap. Two beams were introduced into the Dove prism from opposite ends. The optical image of the two elliptical excitations in the same line is shown in Fig. 5b , where the distance between the centres of two beams were approximately 340 μm. These excitations further created assemblies of Ag nanoparticles at metal–fluid interface (see Supplementary Movie 4 ). Interestingly, when these two assemblies were in close proximity, we found interaction between assemblies leading to a linear chain of nanoparticles between them. Figure 5c shows optical image (after rejecting the laser light) of the two plasmonic assemblies, with a thin line of Ag nanoparticles between them. We also observed similar kind of Ag nanoparticle linear-chains when two assemblies were created in an anti-parallel geometry (see Fig. 5d ). The resulting nanoparticle assembly is shown in Fig. 5e . As the assemblies are now closer (compared with the case shown in Fig. 5c ), the nanoparticle bridge formed is thicker in size. It is to be noted that all this manipulation discussed herein is at the metal–fluid interface. If the excitation beam was switched-off, the entire nanoparticle assembly re-dispersed into the solution. This method is reversible over multiple cycles, and can be an excellent preamble to create dynamic assembly of nanoparticles at metal–fluid interface, and can be further harnessed for large-area, dynamic, optical lithography of nanoscale objects. Figure 5: Interaction between dynamic assemblies of plasmonic nanoparticles at metal–fluid interface. ( a ) Schematic representation of dual assembly of Ag nanoparticles on Au film coupled to a prism: green lines are the two laser beams of 532 nm introduced at two opposite ends of the prism. Black arrows indicate the direction of the laser beams (see Supplementary Movie 4 ). Optical images of dual laser excitation in b collinear geometry with opposite k-vectors and ( d ) anti-parallel geometries with opposite k-vectors. ( c ) and ( e ) are optical images (532 nm-rejected) of Ag nanoparticles assembly due to excitation in shown in b and d , respectively. A thin line of nanoparticles bridging the two assemblies is evident. Note that all these assemblies are at metal–fluid interface, and hence can be further manipulated to achieve dynamic lithography. Scale bar, 100 μm for both ( c ) and ( e ). Full size image We have used an unstructured metal film and plasmonic nanoparticles to form a sensitive molecular detection platform. The sample preparation was easy to reproduce, and can be readily integrated with any microfluidic device. There are situations in microfluidics where one needs to control mixing of molecules and/or nanoparticles for a brief period of time. By using our method, one can assemble nanoparticles for a short instance of time, spectrally probe a mixing reaction and release them back into the solution. This capability to trap, probe and release nanoparticles in a controlled way, especially using optical means, will have implications in driving optofluidic chemical and biochemical reactors. It is to be noted that our methodology is not restricted to metal nanoparticles alone. One can trap two different kinds of samples, such as biological cells and nanoparticles in separate traps, and bring them together in close proximity to obtain a mixture. As assembly and probing is done through optical means, one can also utilize the same optical fields to catalyze photochemical reactions. To conclude, we show how plasmon-assisted assembly and SM-SERS can be achieved with a single evanescent-wave excitation on an unstructured metal film. Such dual-function of plasmons at metal–fluid interface can have relevance in trace detection of molecules at interface without having to structure the metal surface. Furthermore, on the same platform, we have shown how nanoparticles can be reversibly assembled and manipulated with ease. This is also unique method to prepare and optically manipulate SERS substrates at metal–fluid interface that is sensitive enough to detect single-molecule spectroscopic signatures. Interestingly, when we used two excitation beams in our experiments, we could create interacting nanoparticle assemblies. The cross-talk between the assemblies led to the formation of a nanoparticle bridge between the optical potentials paving a new way to assemble nanostructure at metal–fluid interface. We envisage that interacting optical potential can be further harnessed in large-area dynamic lithography of nanoparticles at metal–fluid interface. Such capability will of course find tremendous use in micro- and nano-plasmofluidic applications, where plasmonic fields can drive, trap and probe nanoscale objects. Preparation of metal thin films Glass coverslip was washed by acetone followed by drying was used for deposition of metal films. Direct current (DC) sputtering technique was employed to deposit 40 nm thick gold or silver on glass coverslip at a rate of 0.1 Å s −1 in argon atmosphere. Preparation of metallic nanoparticles Silver and gold nanoparticles were synthesized by citrate reduction procedure [61] . Ag nanoparticles: 250 ml, 5.3 × 10 −4 M aqueous solution of AgNO 3 was heated and brought to boiling using a magnetic stirrer cum hot plate. Then 5 ml of 1% sodium citrate solution was added while stirring the solution and kept for ~\n1 h. Au nanoparticles: 250 ml, 6.7 × 10 −4 M aqueous solution of HAuCl 4 was brought to boiling using magnetic stirrer cum hot plate. Then 20 ml of 1% sodium citrate solution was added while stirring the solution and kept for ~\n1 h. Ag@Au nanoparticles: Ag@Au nanoparticles were prepared by seed-growth method [44] , using Ag colloids as seeds. Ag colloid solution of 12.5 ml was diluted with 10 ml of Mili-Q water, and 2.5 ml of 6.25 × 10 −3 M NH 2 OH, HCl and 2.5 ml of 4.65 × 10 −4 M HAuCl 4 were added drop wise (ca 2 ml min −1 ) by two separate pipettes with vigorous stirring. The amount of HAuCl 4 , here, governs the Au to Ag ratio. The stirring was continued for 45 min to complete reduction. The Ag@Au nanoparticles were characterized by ultraviolet–visible spectrometer and transmission electron microscope (Tecnai F20, FEI, 200 kV). Sample preparation for SM-SERS experiments Ag@Au nanoparticles were mixed with two dye molecules, nile blue chloride (NB) and rhodamine 6G chloride (R6G) such that the final concentration of dye molecules is 5 nM and 80 μl of such solution was drop casted on glass coverslip pre-deposited with 40-nm thick silver film. A series of spectra were collected with an acquisition time of 0.1 s each, with a refresh time of 1 s between each acquisition. The laser power used was 20 mW before entering the prism. The signal collection spot was fixed to 5 μm by keeping the confocal hole size as 400 μm. Water immersion × 60 OBL (NA=1) was used for signal collection. Note that there were no external aggregating agents used. For concentration-dependent SERS measurements, all the parameters of the experiments were held same as SM-SERS studies except the molecular concentration. The probability distribution data for higher bi-analyte concentration and other details for ultra-low concentration measurements can be found in Supplementary Fig. 7 and Supplementary Note 3 . Sample preparation for trapping experiment For nanoparticle trapping experiments, two metal films (gold and silver) and three nanoparticles (Ag, Ag@Au and Au) were used for comparative study. 80 μl colloidal solutions were dropped on to the metal film to observe the trapping phenomena. The colloids were diluted in water such that the number of nanoparticles per ml remained almost same for every colloidal solutions used in different experiments. The metal film thickness was kept constant to 40 nm for both silver and gold films. The LASER power was kept 37 mW before entering the prism throughout all trapping experiments. Videos/images were collected using × 4 OBL (NA=0.13). How to cite this article: Patra, P.P. et al. Plasmofluidic single-molecule surface-enhanced Raman scattering from dynamic assembly of plasmonic nanoparticles. Nat. Commun. 5:4357 doi: 10.1038/ncomms5357 (2014).